A modern ionotropic glutamate receptor with a K+selectivity signature sequence Glutamate is the major excitatory neurotransmitter in the mammalian central nervous system and gates non-selective cation channels. The origins of glutamate receptors are not well understood as they differ structurally and functionally from simple bacterial ligand-gated ion channels. Here we report the discovery of an ionotropic glutamate receptor that combines the typical eukaryotic domain architecture with the 'TXVGYG' signature sequence of the selectivity filter found in K + channels. This receptor exhibits functional properties intermediate between bacterial and eukaryotic glutamate-gated ion channels, suggesting a link in the evolution of ionotropic glutamate receptors. Rapid signal transduction in the central nervous system of vertebrates relies on the neurotransmitter glutamate (Glu) and ionotropic glutamate receptors (iGluRs) [1] . Historically, iGluRs were grouped according to their responses to the small molecule agonists AMPA (α-amino-3-hydroxyl-5-methyl-4-isoxazolepropionic acid; GluA1-A4), kainate (GluK1-K5) and NMDA ( N -methyl- D -aspartate; GluN1, GluN2A-D and GluN3A and B). The origins of iGluRs form the basis of their functional and structural diversity but are currently not understood [2] , [3] , [4] . Simple bacterial iGluRs, such as GluR0 from Synechocystis , presumably arose from the fusion of periplasmic binding proteins and K + channels ( Fig. 1a , left) [4] , [5] , [6] , [7] . GluR0 differs in several major ways from its metazoan and plant homologues [5] . Structurally, it has only two transmembrane (TM) segments, instead of three, and no N-terminal domain (NTD; Fig. 1a ). Functionally, it distinguishes itself from the non-selective cation permeation of iGluRs in being K + -selective because of its pore loop (P-loop), which contains the 'TXVGYG' signature sequence of the K + channel selectivity filter ( Fig. 1b ). Pharmacologically, GluR0 is activated by amino acids other than Glu but not by classical iGluR agonists. 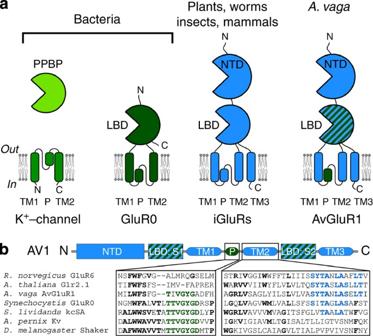Figure 1: Origins of ionotropic glutamate receptors (iGluRs). (a) Transmembrane (TM) and domain organization of iGluRs, AvGluR1 and proteins resembling bacterial ancestors. Colour shading is based on sequence identities of individual domains (also seeSupplementary Table S1). (b) Sequence alignment of pore loop and TM2 for AvGluR1, iGluRs from mammals and plants, and GluR0 and K+channels. Residues found in at least three sequences are highlighted in bold. Colours highlight conserved motifs. NTD, N-terminal domain; PPBP, periplasmic binding protein. Figure 1: Origins of ionotropic glutamate receptors (iGluRs). ( a ) Transmembrane (TM) and domain organization of iGluRs, AvGluR1 and proteins resembling bacterial ancestors. Colour shading is based on sequence identities of individual domains (also see Supplementary Table S1 ). ( b ) Sequence alignment of pore loop and TM2 for AvGluR1, iGluRs from mammals and plants, and GluR0 and K + channels. Residues found in at least three sequences are highlighted in bold. Colours highlight conserved motifs. NTD, N-terminal domain; PPBP, periplasmic binding protein. Full size image The complex domain architecture shared by eukaryotic iGluRs ( Fig. 1a , middle) suggests a common eukaryotic ancestor [2] , [8] that may merge elements of GluR0, similar to the K + selectivity filter, with those of iGluRs, similar to the NTD or C terminus. In this study, we report the discovery and functional characterization of AvGluR1, which is the first eukaryotic iGluR with the complex architecture of vertebrate iGluRs and the signature sequence of the K + channel selectivity filter. Domain organization and function seem to indicate that AvGluR1 represents the 'transitional stage' between bacterial and vertebrate iGluRs. Identification and structure We searched the eukaryotic protein database of the National Center for Biotechnology Information with artificial sequences that combined a mammalian ligand-binding-domain (LBD) and C terminus (either from GluK2, GluA2 or GluN1) with a K + selectivity filter (from GluR0, Methods). The only protein returned by these searches that aligned to iGluRs over all domains was a putative iGluR from the freshwater bdelloid rotifer Adineta vaga , a remarkable model organism for asexual reproduction and horizontal gene transfer, whose genome has been partially sequenced [9] . We termed this uncharacterized iGluR as AvGluR1. The domain organization of AvGluR1 mirrors that of eukaryotic iGluRs ( Fig. 1a , right). It features the 'SYTAXLA' motif in TM2 that is conserved in all known eukaryotic iGluRs [3] ( Fig. 1b ) but contains a 'TXVGYG' motif in its P-loop, as in GluR0 and K + channels. Consequently, the P-loop of AvGluR1 aligns most closely to that of K + channels, whereas the remainder of the TM domain resembles that of iGluRs ( Supplementary Table S1 ). The LBD exhibits weaker similarity to both eukaryotic iGluRs and GluR0, but an arginine residue that contacts the α-carboxyl group of the ligand in all mammalian iGluRs (for example, R523 in GluK2) is conserved in AvGluR1 (R546) and so is an acidic residue contacting the α-amino group (E738 in GluK2), which is an aspartic acid in AvGluR1 (D744) and in all NMDA receptors ( Supplementary Fig. S1 ). Residues contacting the γ-carboxyl of Glu are not conserved in AvGluR1 (for example, T690 in GluK2 is A704 in AvGluR1, similarly in GluN3A and B but in no other iGluR) and AvGluR1 can gate upon binding amino-acid ligands other than Glu (see below). There is low conservation of the NTD of GluK2 compared with AvGluR1 ( Supplementary Table S1 ) and with other lower invertebrates (data not shown), except for two marked cysteine residues ( Supplementary Fig. S1 ) that stabilize the NTD in all mammalian iGluRs [10] . Finally, AvGluR1 has a C terminus that is 43 amino acids in length, the sequence of which shows no homology to any known protein. Similarly, no homologues are found for the C-termini of many iGluRs of lower invertebrates (data not shown). Functional characterization When we expressed AvGluR1 in Xenopus laevis oocytes, we recorded large currents in response to Glu perfusion ( Figs 2a and 3a ). Similar to GluR0, AvGluR1 was gated by Glu with high potency (EC 50 =4.0 μM; 95% confidence interval 0.8–20.0 μM, N =7; Fig. 2b ). AvGluR1 was also gated by several other amino acids, including aspartate, serine, glutamine and, very weakly, by glycine ( Fig. 2a ). Glycine had no effect on the response to Glu ( Supplementary Fig. S2 ). These amino acids do not gate AMPA and kainate receptors but serve as agonists of NMDA receptors [5] , [11] , [12] , [13] . AvGluR1 was also gated by iGluR agonists kainate and AMPA ( Fig. 2a and Supplementary Fig. S3 ), as observed for mammalian receptors, but not for GluR0 [5] , [11] , [12] , [14] . For aspartate and kainate, the difference in agonist response seems to be due to a shift in potency as the currents extracted from the fit at the EC 50 concentration are in the same range as for Glu ( Supplementary Fig. S3 ). 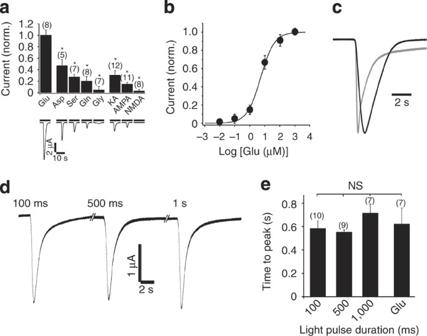Figure 2: Agonist specificity and slow gating of AvGluR1. (a) Agonist specificity measured for 1-mM agonist concentration. Traces of single-cell responses to various agonists (bottom). Bar graphs show average current amplitudes±s.e.m. for multiple cells (top). *F-test analysis of variance showed that agonist responses are significantly different at the 1% level (P<10−10).Post hocanalysis using the Tukey–Kramer method showed that the response to Glu is different from that of all other agonists at the 1% significance level (P<0.0001 for each pairwise comparison). (b) Peak AvGluR1 response to 15 s application of Glu at various concentrations (mean±s.e.m. from seven oocytes). Data were fit as described in the Methods section (EC50=4.0 μM, 95% confidence interval 0.8–20.0 μM,h=1.0,n=7). In (a) and (b), agonists were applied at 3-min intervals to allow recovery from desensitization. (c) Normalized currents of GluK2 (grey trace) and AvGluR1 (black trace) elicited by prolonged 1-mM Glu application reveal slow activation of AvGluR1. (d) Currents elicited by 20-μM MNI-caged-L-glutamate released by light pulses of different durations also rise slowly. (f) Time to peak of AvGluR1 currents elicited by Glu uncaging or perfusion (NS indicates no statistically significant differences using Student'st-test,P≥0.2). In (a) and (e), number of observations is shown in parentheses. NS, not significant. Figure 2: Agonist specificity and slow gating of AvGluR1. ( a ) Agonist specificity measured for 1-mM agonist concentration. Traces of single-cell responses to various agonists (bottom). Bar graphs show average current amplitudes±s.e.m. for multiple cells (top). *F-test analysis of variance showed that agonist responses are significantly different at the 1% level ( P <10 −10 ). Post hoc analysis using the Tukey–Kramer method showed that the response to Glu is different from that of all other agonists at the 1% significance level ( P <0.0001 for each pairwise comparison). ( b ) Peak AvGluR1 response to 15 s application of Glu at various concentrations (mean±s.e.m. from seven oocytes). Data were fit as described in the Methods section (EC 50 =4.0 μM, 95% confidence interval 0.8–20.0 μM, h =1.0, n =7). In ( a ) and ( b ), agonists were applied at 3-min intervals to allow recovery from desensitization. ( c ) Normalized currents of GluK2 (grey trace) and AvGluR1 (black trace) elicited by prolonged 1-mM Glu application reveal slow activation of AvGluR1. ( d ) Currents elicited by 20-μM MNI-caged- L -glutamate released by light pulses of different durations also rise slowly. ( f ) Time to peak of AvGluR1 currents elicited by Glu uncaging or perfusion (NS indicates no statistically significant differences using Student's t -test, P ≥0.2). In ( a ) and ( e ), number of observations is shown in parentheses. NS, not significant. 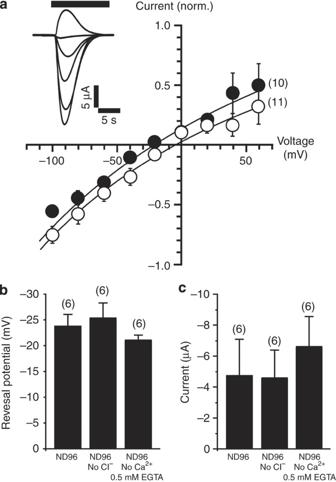Figure 3: Ion selectivity of AvGluR1. (a) Current–voltage relationship of AvGluR1 in Na+(solid circles) and K+(open circles) extracellular solution. The reversal potential shifts by 19.7 mV from −24.3 to −2.5 mV. Inset: Representative Glu-gated currents at −100, −80, −60, −40, −20 to 0 mV in Na+extracellular solution. (b,c) Reversal potentials (b) and current amplitudes (c) in normal extracellular ND96 solution (containing 1.8-mM Ca2+), Ca2+-free ND96 (zero added extracellular Ca2+with 0.5-mM EGTA) and Cl−-free ND96 (Cl−is replaced with gluconate). In (b) and (c) number of observations shown in parentheses and no statistically significant differences were observed using Student'st-test (P≥0.4). Full size image Figure 3: Ion selectivity of AvGluR1. ( a ) Current–voltage relationship of AvGluR1 in Na + (solid circles) and K + (open circles) extracellular solution. The reversal potential shifts by 19.7 mV from −24.3 to −2.5 mV. Inset: Representative Glu-gated currents at −100, −80, −60, −40, −20 to 0 mV in Na + extracellular solution. ( b , c ) Reversal potentials ( b ) and current amplitudes ( c ) in normal extracellular ND96 solution (containing 1.8-mM Ca 2+ ), Ca 2+ -free ND96 (zero added extracellular Ca 2+ with 0.5-mM EGTA) and Cl − -free ND96 (Cl − is replaced with gluconate). In ( b ) and ( c ) number of observations shown in parentheses and no statistically significant differences were observed using Student's t -test ( P ≥0.4). Full size image AvGluR1 currents activated slowly but exhibited full desensitization to prolonged agonist application ( Figs 2a,c and 3a ). The slow activation of AvGluR1 resembles the behaviour of GluR0, and is distinct from the rapidly activating iGluRs ( Fig. 2c ), whereas the full desensitization resembles the behaviour of iGluRs but differs from GluR0, which only desensitizes partially [5] . Slow activation was also observed when agonist was presented by photolysis of caged- L -Glu ( Fig. 2d,e ). Finally, despite having a K + channel type selectivity filter sequence, AvGluR1 exhibited a poor selectivity for K + over Na + , similar to that of vertebrate iGluRs. Analysis with the Goldman–Hodgkin–Katz equation indicates a P Na+ / P K+ permeability ratio of 0.3 (versus 0.01 for GluR0 and 0.8 for GluK2 [5] , [15] ; Fig. 3a and Supplementary Fig. S4 ). To test for Ca 2+ permeability, we compared currents recorded in normal extracellular solution (containing 1.8-mM Ca 2+ ) and in the absence of Ca 2+ (zero added extracellular Ca 2+ with 0.5-mM EGTA). Neither current amplitude nor reversal potential differed between these conditions ( Fig. 3b,c ). Moreover, the Ca 2+ -activated Cl − channels of Xenopus oocytes [16] did not contribute to the current, as replacing external Cl − did not modify either Glu-evoked current amplitude or reversal potential of AvGluR1. These data indicate that the channel has little or no permeability to Ca 2+ ( Fig. 3a,b ). Together, amino-acid sequence, domain organization and function indicate that AvGluR1 represents a functional intermediate between GluR0 and iGluRs. Phylogenetic analysis To further examine the relationship between AvGluR1 and iGluRs, we performed a phylogenetic analysis of 251 iGluRs sampled from bacteria, plants and animals ( Supplementary Tables S2 and S3 ). In particular, we collected all iGluR-like proteins from the few early branching animals that have such sequences (for example, Trichoplax adhaerens , the cnidarian Nematostella vectensis or the mollusk Aplysia californica ). Phylogeny was inferred using several methods, including maximum likelihood (ML) with RAxML [17] . In the ML phylogeny ( Fig. 4 ), AvGluR1 branches out early compared with all other metazoan iGluRs with bootstrap support of 77 and 85%. Trees built using different ML methods and neighbour joining yielded the same branching order and similar bootstrap support, as did trees built on a larger data set automatically collected by FlowerPower [18] , and if the GYG sequence in AvGluR1 was replaced by three consecutive glutamines to mimic non-NMDA iGluRs (data not shown). This branching order supports the functional analysis and suggests that AvGluR1 represents a transitional stage between bacterial and metazoan iGluRs. In particular, the phylogenetic analysis allows excluding the possibility that AvGluR1 arose from the secondary acquisition of the 'TXVGYG' sequence by a rotifer iGluR. In such a re-evolution scenario, the overall sequence of AvGluR1 should resemble that of iGluRs from animals that started to develop independently before and after rotifers. Phylogenetic analysis would then place AvGluR1 deep within the animal part of the tree, which is not observed. 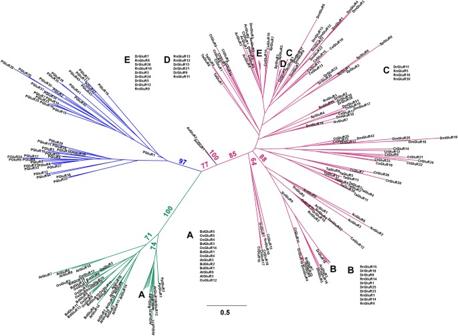Figure 4: Maximum likelihood (ML) tree of AvGluR1 and ionotropic glutamate receptors (iGluRs). A total of 251 iGluR sequences were collected from all three kingdoms of life and the ML tree was constructed as described in the Methods section. Bootstrap support values are shown at the major branches. Taxa and branches are colour coded with bacteria in blue, plants in green, animals in magenta and AvGluR1 and AvGluR2 in purple. A–E are expansions of lists of genes that are too packed to be seen in the branch cartoon. The scale bar refers to evolutionary distance inferred by the RAxML algorithm. Figure 4: Maximum likelihood (ML) tree of AvGluR1 and ionotropic glutamate receptors (iGluRs). A total of 251 iGluR sequences were collected from all three kingdoms of life and the ML tree was constructed as described in the Methods section. Bootstrap support values are shown at the major branches. Taxa and branches are colour coded with bacteria in blue, plants in green, animals in magenta and AvGluR1 and AvGluR2 in purple. A–E are expansions of lists of genes that are too packed to be seen in the branch cartoon. The scale bar refers to evolutionary distance inferred by the RAxML algorithm. Full size image The origins of iGluRs are mysterious [2] , [3] , [4] . Our own database search (Methods) confirmed that iGluRs are absent from basal eukaryotes, such as fungi, protozoa or the sponge Amphimedon queenslandica [2] , [19] . We cloned and characterized an iGluR, the amino-acid sequence, domain organization and function of which resembles the missing intermediate between bacterial and eukaryotic iGluRs. In the A. vaga genome, the gene coding for AvGluR1 is located near transposable elements [9] and we cannot exclude the fact that it originates from horizontal gene transfer [20] . The existence of bacterial ion channels with an LBD but without K + selectivity motif raised the question as to which class of proteins developed into iGluRs [21] . Our findings suggest that iGluRs evolved by addition of an NTD and TM3 to a GluR0-like protein that contained a 'TXVGYG' motif. These new domains endow new functionalities to iGluRs, in that NTDs provide for sub-type-specific assembly and modulation of gating, whereas the third TM helix locates the C terminus intracellularly for sorting, binding to the cytoskeleton and modulation [1] . The promiscuous agonist binding of AvGluR1 is divergent from typical AMPA, kainate or NMDA receptors and rather resembles that of chemosensory receptors in single cell organisms and sensory cells of multicellular organisms [22] . Indeed, iGluR-like chemosensors that lack an NTD were recently identified in the fruit fly, and it will be interesting to see how these proteins and AvGluR1 accommodate a chemically diverse spectrum of ligands. The low conservation of the NTD and C terminus of AvGluR1 may not be surprising as this receptor likely serves different roles than modern neurotransmitter receptors for which cytosolic association and modulation are crucial. The identification of AvGluR1 and voltage-sensing phosphatases [23] thus re-emphasizes the fact that exotic invertebrates offer a repertoire of novel proteins that remain to be discovered. Uniprot accession numbers The following sequences were used for the alignment of Figure 1 and Supplementary Figure S1 (Uniprot identifiers in parentheses): Rattus norvegicus GluK2 (P42260), Arabidopsis thaliana Glr2.1 (O04660), Synechocystis GluR0 (P73797), Streptomyces lividans KcsA (P0A334), Aeropyrum pernix K v (Q9YDF8) and Drosophila melanogaster Shaker (P08510). Sequences were aligned using Muscle 3.8 (ref. 24 ) with the default parameters. AvGluR1 identification and bioinformatics AvGluR1 (Uniprot identifier B3G447) was identified in the National Center for Biotechnology Information non-redundant protein database, using a search with PHI-Blast. The primary query sequence was a chimeric protein of GluK2 (from R. norvegicus , LBD, TM3 and C terminus, residues 426–556 and 658–908) and GluR0 (from Synechocystis PCC 6803, pore domain, residues 154–246). Residues are numbered beginning with the start-methionine. The query was limited to eukaryotes (taxonomy ID 2759) and the PHI (pattern hit initiated) pattern [TVIL]-G-[YF]-G-[DFLYGHKARN] that covers the K + selectivity filter of a majority of K + channels [25] . As of 25 August 2010, AvGluR1 is the highest ranking hit for this query (27% identity) and the only hit aligning close to the entire length of the protein. Identical queries using the LBD, TM3 and C terminus taken from the GluA2 AMPA receptor (from R. norvegicus , Uniprot identifier Q9R174, residues 409–539 and 644–883) or the GluN1 NMDA receptor (from R. norvegicus , Uniprot identifier P35439, residues 413–555 and 654–938) also yielded AvGluR1 as the highest ranking hit. Preparation of expression constructs The a-splice isoform of GluK2 was obtained from K. Partin (Colorado State University, Fort Collins, CO) and cloned into pGEM-HE. Genomic DNA of A. vaga was a kind gift from E. Gladyshev and I. Arkhipova (Marine Biology Laboratory, Woods Hole, MA and Harvard University, Cambridge, MA). Forward (TATCCCGGGCACCATGAGAATATTTCGAGAAAACATCTCGTG) and reverse (ATATCTAGATTATGCAATGATTTGTGATATAGTAGACGAAG) oligonucleotide primers for polymerase chain reaction (PCR) included Xma I and Xba I restriction sites for subcloning into pGEM-HE. PCR reaction parameters were as follows: One cycle at 95 °C for 60 s; 32 cycles at 95 °C for 30 s, at 56 °C for 30 s and at 72 °C for 180 s; and one cycle at 95 °C for 10 min. Several independent PCR reactions yielded the same AvGluR1 sequence that differs from that deposited in genome sequencing in 26 positions (Accession Codes). RNA preparation and electrophysiology RNA was transcribed using a mMessage mMachine T7 transcription kit (Ambion). Surgically extracted X. laevis oocytes were injected with 5 ng of RNA in 50-nl volume. Cells were incubated in ND-96 solution (96-mM NaCl, 2-mM KCl, 1.8-mM CaCl 2 , 1-mM MgCl 2 , 50-mg ml −1 gentamicin, 2.5-mM sodium pyruvate and 5-mM Hepes, pH 7.4) at 18 °C for 12–36 h before experiments. Cells expressing GluK2 were pretreated with concanavalin-A. The two-electrode voltage-clamp technique was used at room temperature with a Dagan CA-1B amplifier, Digidata-1440A data acquisition board and pClamp10 software. Oocytes were placed in a perfusion dish and data were recorded in ND-96 recording solution without antibiotics. For uncaging the MNI-caged-Glu (4-methoxy-7-nitroindolinyl-caged- L -glutamate), illumination was carried out with a 150-W xenon lamp through a Nikon Diaphot inverted microscope with a ×20 0.75 NA fluorescence objective (Nikon). Illumination time was defined by a Uniblitz shutter (Vincent Associates) controlled by the Digidata-1440 board and pClamp10 software package (Axon Instruments). Data analysis To estimate relative permeabilities of Na + and K + , we analysed reversal potentials using the simplified Goldman–Hodgkin–Katz voltage equation, P Na+ / P K+ =exp(Δ E rev F / RT ), where Δ E rev is the reversal potential difference between Na + and K + , F is Faraday's constant, R is the gas constant and T is temperature and after correction for liquid junction potentials. To determine the EC 50 ( Fig. 2 and Supplementary Fig. S3 ), dose–response data were fit in SigmaPlot with the Hill equation I = x h /( x h +EC 50 h ), where I represents the normalized current, x represents concentration and h is the Hill coefficient. iGluRs in archaea and unicellular eukaryotes To identify iGluRs in archaea and unicellular eukaryotes, we searched the non-redundant protein database of the National Center for Biotechnology Information with Blast. We used GluK2 from R. norvegicus as the query sequence and limited the search to archaea (2157), fungi (4751), monosiga (81525), diatoms (2836), alveolata (33630), trypanosome (5690) and dictyostelium (5782; numbers in parentheses are taxonomy identifiers). As of 25 August 2010, highest-ranking hits were K + channels or completely unrelated proteins with E -values near zero. No proteins that contained an iGluR-like LBD and TM domain could be identified. Phylogenetic analysis Using Blast searches, we identified 251 iGluR-like proteins in bacteria, plants and animals, with special attention to early branching eukaryotes ( Supplementary Table S2 ). For these organisms, we collected all proteins that aligned to AvGluR1 or GluK2 over the pore and LBD. This data set included iGluRs that were identified previously, as well as sequences that have not yet been annotated ( Supplementary Table S3 ). This search also revealed AvGluR2 (Uniprot identifier B3G464), an A. vaga protein that features the TXVGYG-pore motif and shares 53% sequence identity with AvGluR1. Sequences were aligned with Muscle [26] . Gaps and the N- and C-terminal domains only found in eukaryotic proteins were manually removed. Phylogenetic analysis was primarily performed with the ML method and RAxML 7.2.6 (ref. 17 ). A total of 20 ML searches were conducted to find the best ML tree ( Fig. 4 ) and branch support was assessed with 100 bootstrap replicates. We observed the same branching order of AvGluR1 in trees that were built with different amino-acid substitution matrices, through neighbour joining with BioNJ [27] and based on a data set of 606 proteins automatically collected with FlowerPower [18] , followed by neighbour joining. Accession codes: Sequences of AvGluR1 and AvGluR2 have been deposited in GenBank under accession codes HQ901600 and HQ901601 . How to cite this article: Janovjak, H. et al . A modern ionotropic glutamate receptor with a K + selectivity signature sequence. Nat. Commun. 2:232 doi: 10.1038/ncomms1231 (2011).